Rapid and adaptive evolution of MHC genes under parasite selection in experimental vertebrate populations The genes of the major histocompatibility complex are the most polymorphic genes in vertebrates, with more than 1,000 alleles described in human populations. How this polymorphism is maintained, however, remains an evolutionary puzzle. Major histocompatibility complex genes have a crucial function in the adaptive immune system by presenting parasite-derived antigens to T lymphocytes. Because of this function, varying parasite-mediated selection has been proposed as a major evolutionary force for maintaining major histocompatibility complex polymorphism. A necessary prerequisite of such a balancing selection process is rapid major histocompatibility complex allele frequency shifts resulting from emerging selection by a specific parasite. Here we show in six experimental populations of sticklebacks, each exposed to one of two different parasites, that only those major histocompatibility complex alleles providing resistance to the respective specific parasite increased in frequency in the next host generation. This result demonstrates experimentally that varying parasite selection causes rapid adaptive evolutionary changes, thus facilitating the maintenance of major histocompatibility complex polymorphism. The immunogenes of the major histocompatibility complex(MHC) show the most outstanding genetic polymorphism in jawed vertebrates [1] , [2] . The MHC is a multigene family that has a decisive role in controlling the vertebrate adaptive immune system by presenting self- and parasite-derived peptides to T cells [3] . To counteract parasitic attacks, new allele combinations of hosts' resistance immunogenes should be favoured every generation. As the accumulation of new beneficial mutations is slow, standing genetic variation can become crucial for rapid adaptation. With their well-characterized function and exceptional diversity, MHC genes thus represent excellent candidates to investigate the mechanisms for the maintenance of standing genetic variation, described as one of the greatest evolutionary puzzles [2] , [4] , [5] . A series of hypotheses propose that MHC polymorphism could be maintained by a form of balancing selection, mediated by parasites and pathogens through heterozygote advantage, negative frequency-dependent selection, and spatially or temporally varying parasite pressure (for review, see refs 2 , 6 , 7 , 8 ). Although distinct, those three mechanisms are not mutually exclusive, and can act in synergy. Mathematical models showed that heterozygote advantage is not sufficient to maintain MHC polymorphism alone [9] , [10] , but may contribute to it [11] . Under negative frequency-dependent selection, a rare resistance allele should increase in frequency over time [12] , [13] . This increase may be due to a direct selective advantage through allele-specific parasite resistance [14] , and may be indirectly amplified by mate choice, where females favour mating with males carrying the resistance allele [15] , [16] , [17] . In the following generations, a new parasite species or genotype may become frequent and, as a consequence, a different host MHC allele may provide resistance and thus should increase in frequency. This phenomenon represents an adaptive allele frequency shift. Both negative frequency-dependent selection and temporally varying parasite-mediated selection can produce such adaptive frequency shifts of resistance MHC alleles with selection re-occurring with every new predominant parasite species, or genotype in time or space. Annual population surveys of great reed warblers [18] , house finches [19] , three-spined sticklebacks [20] and Soay sheep [21] represent observational examples of variation in MHC allele frequencies between successive generations. Additionally, variation of MHC allele pools across neighbouring populations has been recorded for several species, consistent with spatially varying parasite pressures (for examples, see refs 22 , 23 ). Probably because MHC is restricted to vertebrates where experimental testing at the population level is demanding, experimental proof of rapid adaptive frequency shift is still awaited [5] . Such a phenomenon would represent the necessary pre-requisite for evolutionary dynamics, where the host needs to rapidly adapt to constantly changing parasite pressures (that is, the Red Queen dynamics [24] , [25] ), and provide evidence for variable parasite pressure as a mechanism for maintaining MHC polymorphism. In this study, genetically identical experimental populations of three-spined sticklebacks were each selected for resistance to one of two different sympatric parasite species, and MHC allele frequencies were tracked between two generations. If an allele frequency shift occurred and was adaptive, those MHC alleles that increased in frequency should be the ones that provided resistance against the particular selecting parasite. Because these replicated experimental populations were each exposed to one of two different parasite species, distinct directional selection should lead to the increase in frequency of at least two different resistance MHC alleles. And indeed, we found that only those MHC alleles providing resistance to the respective specific parasite increased in frequency in the next host generation. No consistent frequency changes were observable at neutral markers suggesting the adaptive significance of such frequency shifts independently of any demographical events. Mortality was not responsible for the increase in frequency of those MHC alleles. Therefore, fitter individuals must have reproduced more and/or females may have been able to choose preferentially males carrying those resistance MHC alleles. Parasite mediated selection After allowing the experimental G1 fish to mate and reproduce naturally under selection by one of the two parasites, we tested for the evolution of higher resistance by exposing fish of the next generation (G2) to either the same, or to the other, parasite species as their parents. G2 fish turned out to be more resistant to the parasite that their parents had been exposed to, than the other in both treatments (Mixed effect models, Anguillicoloides crassus , t -value=−2.02, d.f.=392, P =0.042; Camallanus lacustris , t -value=2.93, d.f.=385, P =0.021 ( Fig. 1 ; Supplementary Fig. S1 )). 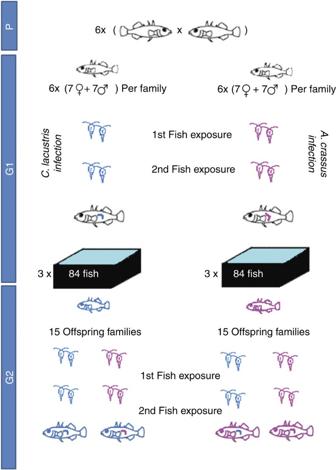Figure 1: Experimental design. Twelve randomly caught fish (parental generation, P) were crossed to obtain six laboratory-bred families (Generation 1, G1). A total of 6 families contributed equally to 6 experimental populations (7 males & 7 females per family per population, 84 fish per population, 504 fish in total). Three populations were exposed to laboratory-bred copepods infected with the nematodeA. crassus(in total over the 2 generations,N=18,000 copepods andN=49,600 parasite larvae) and 3 were exposed to laboratory-bred copepods infected with the nematodeC. lacustris(in total,N=20,000 copepods andN=127,000 parasite larvae). After natural reproduction in the artificial ponds, clutches were collected and fry-reared under standard conditions. Each clutch was then split into two equal groups and fish (N=450 per parental treatment, Generation 2, G2) were exposed either to the same parasite as their parents or the alternative parasite. Blue is used for copepods and fish exposed toC. lacustris, and purple is used for copepods and fish exposed toA. crassus. Figure 1: Experimental design. Twelve randomly caught fish (parental generation, P) were crossed to obtain six laboratory-bred families (Generation 1, G1). A total of 6 families contributed equally to 6 experimental populations (7 males & 7 females per family per population, 84 fish per population, 504 fish in total). Three populations were exposed to laboratory-bred copepods infected with the nematode A. crassus (in total over the 2 generations, N =18,000 copepods and N =49,600 parasite larvae) and 3 were exposed to laboratory-bred copepods infected with the nematode C. lacustris (in total, N =20,000 copepods and N =127,000 parasite larvae). After natural reproduction in the artificial ponds, clutches were collected and fry-reared under standard conditions. Each clutch was then split into two equal groups and fish ( N =450 per parental treatment, Generation 2, G2) were exposed either to the same parasite as their parents or the alternative parasite. Blue is used for copepods and fish exposed to C. lacustris , and purple is used for copepods and fish exposed to A. crassus . Full size image Trans-generational MHC frequency changes Is this resistance effect related to specific MHC alleles? In the original lake population, MHC class IIβ genes occur in several copies, linked in distinct haplotypes with one-to-three different alleles achieved either through a variable number of loci, or identical alleles on paralogous loci [26] . In our G1 families, 18 different MHC class IIβ variants, linked into 9 haplotypes, were present (sequences are given in Supplementary Table S1 ). Individual MHC genotype diversity ranged from 2-to-5 variants. As expected under our balanced design, MHC diversity did not vary among G1 experimental populations before treatment neither in terms of individual diversity (that is, number of allele per genotype between treatments, Kruskal–Wallis, U =0.58, d.f.=1, P =0.45) nor in terms of haplotype frequencies (analysis of similarity (ANOSIM), R =0.002, P =0.31). After fish were allowed to reproduce under contrasting parasite selection regimes, we found significant differences in MHC haplotype frequencies between treatments in the resulting second generation (G2, N A. crassus =450, N C. lacustris =450, ANOSIM, R =0.033, P =0.001) ( Fig. 2 ; Supplementary Fig. S2 ). As G2 clutches showed less than 2% mortality in the laboratory, during both egg and juvenile stages, these effects probably have arisen from MHC-dependent differences in fecundity and/or attractiveness, and not from differential survival rates. Additionally, treatment effects were observed only at MHC genes and not at neutral microsatellites, where there were no differences between treatments ( Supplementary Table S2 ; Supplementary Fig. S3 ). 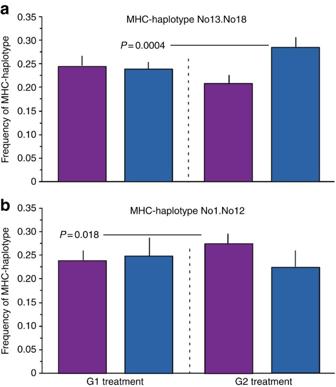Figure 2: MHC Allele frequency shift. Mean (+1 s.e.m.) frequency changes of the resistance haplotypes between the first generation (G1) and the second generation (G2). After fish were allowed to reproduce under contrasting parasite selection regimes, MHC haplotype frequencies vary between treatments in G2 (NA. crassus=450, NC. lacustris=450, ANOSIM,R=0.033,P=0.001). Two MHC haplotypes (No13.No18 and No01.No12) explained 20.3 and 19.6%, respectively, of the variance between parasite treatments. The frequency change between generations was then tracked within each treatment (a) The haplotype No13.No18 increases in frequency (X2=16.58, d.f.=1,P<0.0005) underC. lacustrisselection—a parasite to which it confers resistance. (b) No01.No12 increases in frequency (X2=5.53, d.f.=1,P=0.019) underA. crassusselection, a parasite to which it confers resistance. Frequencies are averaged over replicated experimental ponds. Blue bars represent fish exposed toC. lacustrisand purple bars represent fish exposed toA. crassus. Figure 2: MHC Allele frequency shift. Mean (+1 s.e.m.) frequency changes of the resistance haplotypes between the first generation (G1) and the second generation (G2). After fish were allowed to reproduce under contrasting parasite selection regimes, MHC haplotype frequencies vary between treatments in G2 (N A. crassus =450, N C. lacustris =450, ANOSIM, R =0.033, P =0.001). Two MHC haplotypes (No13.No18 and No01.No12) explained 20.3 and 19.6%, respectively, of the variance between parasite treatments. The frequency change between generations was then tracked within each treatment ( a ) The haplotype No13.No18 increases in frequency ( X 2 =16.58, d.f.=1, P <0.0005) under C. lacustris selection—a parasite to which it confers resistance. ( b ) No01.No12 increases in frequency ( X 2 =5.53, d.f.=1, P =0.019) under A. crassus selection, a parasite to which it confers resistance. Frequencies are averaged over replicated experimental ponds. Blue bars represent fish exposed to C. lacustris and purple bars represent fish exposed to A. crassus . Full size image Adaptive MHC allele frequency shifts Through selection by a given parasite, we expected a resistance haplotype to increase in frequency in G2 and thus to explain a substantial part of the variance in allele frequencies between G1 treatments. Indeed, we found two such MHC haplotypes (No13.No18 and No01.No12; Supplementary Figs S2 and S4 ) explaining 20.3 and 19.6% of the variance between parasite treatments, respectively. Haplotype No13.No18 increased by 19.7% in frequency under C. lacustris selection, whereas haplotype No01.No12 increased by 15.5%, in frequency under A. crassus selection ( Fig. 2 ). As expected under an adaptive haplotype frequency-shift scenario, haplotype No01.No12 conferred resistance against A. crassus whereas No13.No18 conferred resistance against C. lacustris ( Fig. 3 ; Supplementary Table S3 ). There was no interaction between parasite treatment and resistance conferred by the respective MHC haplotype, that is, carrying the resistance alleles always conferred the same advantage against the respective parasite, irrespective of the parasite selecting the parents. This suggests that the haplotype frequency shifted as the result of positive selection and not as the result of change in the resistance function of the respective alleles owing to non-genetic effects, for instance, (Mixed effect models, A. crassus , t -value=−1.52, d.f.=392, P =0.13; C. lacustris , t -value=0.23, d.f.=385, P =0.82; Supplementary Table S3 ). Therefore, these haplotypes should have conferred the respective resistance already in the G1 generation. Indeed G1 fish carrying the haplotypes No13.No18 and No01.No12 were less infected by the respective selective parasites than fish lacking those haplotypes (Mixed effect models, d.f.=196, t -value=−3.34, P =0.001 for A. crassus and No01.No12, d.f=196, t -value=−5.30, P =0.0001 for C. lacustris and No13.No18; Supplementary Table S4 ). 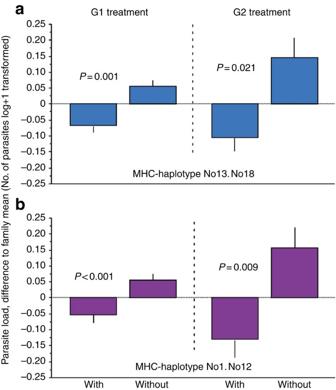Figure 3: Adaptive significance of MHC frequency shifts. Mean (+1 s.e.m.) parasite load as a function of the presence ('with') or absence ('without') of the respective resistance haplotypes (a) No13.No18 and (b) No01.No12 in G1 and G2 generations. Haplotype No13.No18 confers resistance againstC. lacustris(G1,T=−7.4, d.f.=196,P<0.001; G2, d.f.=385,T=−2.61,P=0.009), whereas the haplotype No01.No12 confers resistance againstA. crassus(G1,T=−3.875, d.f.=196,P=0.001, G2T=−2.353, d.f.=392,P=0.021). Parasite data were log+1 transformed to meet normality assumptions. Parasite load is the difference between the average individual infection with and without the resistance haplotype to the average infection within its family. If values are negative, infection is lower than the average family infection whereas, if values are positive, infection is higher than the average family infection. Blue bars represent 13 (out of 15) segregating fish families exposed toC. lacustrisand purple bars represent 12 (out of 15) segregating fish families exposed toA. crassus. Parasites were counted during fish dissection. The other families did not contain individuals both with and without the respective haplotypes and were therefore excluded to guarantee comparability. No13.No18 G1 (N=197) and G2 (N=386). No01.No12 G1 (N=197) and G2 (N=393). Figure 3: Adaptive significance of MHC frequency shifts. Mean (+1 s.e.m.) parasite load as a function of the presence ('with') or absence ('without') of the respective resistance haplotypes ( a ) No13.No18 and ( b ) No01.No12 in G1 and G2 generations. Haplotype No13.No18 confers resistance against C. lacustris (G1, T =−7.4, d.f.=196, P <0.001; G2, d.f.=385, T =−2.61, P =0.009), whereas the haplotype No01.No12 confers resistance against A. crassus (G1, T =−3.875, d.f.=196, P =0.001, G2 T =−2.353, d.f.=392, P =0.021). Parasite data were log+1 transformed to meet normality assumptions. Parasite load is the difference between the average individual infection with and without the resistance haplotype to the average infection within its family. If values are negative, infection is lower than the average family infection whereas, if values are positive, infection is higher than the average family infection. Blue bars represent 13 (out of 15) segregating fish families exposed to C. lacustris and purple bars represent 12 (out of 15) segregating fish families exposed to A. crassus . Parasites were counted during fish dissection. The other families did not contain individuals both with and without the respective haplotypes and were therefore excluded to guarantee comparability. No13.No18 G1 ( N =197) and G2 ( N =386). No01.No12 G1 ( N =197) and G2 ( N =393). Full size image Non-random mortality with regards to the MHC in G1 could explain the observed adaptive frequency shift, if G1 fish lacking the resistance haplotype had higher mortality rate. However, there was no difference in mortality between fish carrying the resistance alleles from those lacking those alleles (Mixed effect models, for A. crassus and No01.No12, d.f.=2, t -value=−0.035, P =0.739; for C. lacustris and No13.No18, d.f=2, t -value=−0.079, P =0.451). Standing genetic variation allows for faster evolutionary changes than the accumulation of new beneficial mutations [4] . The extreme polymorphism of the immune genes of the major histocompatibility complex should thus allow for rapid host evolution given temporally varying parasite selection. Using replicated experimental three-spined stickleback populations, we found that G2 fish were more resistant to the parasite, their parents had been exposed to, than to the other, in both treatments. This happened because different parasites selected for different MHC resistance haplotypes, resulting in adaptive frequency shifts after only one generation. We also found that the two rapidly and positively selected MHC haplotypes did not have a low starting allele frequency. This follows the theory of adaptation from standing genetic variation, where recycling of allelic variants allows faster response than would the spread of beneficial mutations [4] . It also highlights a mechanism where it is neither necessary, nor sufficient for MHC alleles/haplotypes to be rare to increase in frequency. They should become more common starting from any frequency level, driven by the presence of the parasite against which the allele provides resistance; they would not increase from even low frequency if the respective parasite is absent. The tight association between an MHC allele and a parasite is a pre-requisite for initiation of the Red-Queen dynamic. Also, such associations are evidence for the role of diversifying parasite-mediated selection on the maintenance of MHC polymorphism. The two parasites selected consistently across replicates for two different MHC haplotypes, which demonstrates the ability of MHC to efficiently facilitate resistance to individual parasite species. As populations are usually confronted with multiple parasite or pathogen infections in time and space, parasite-mediated selection should maintain higher MHC diversity in natural populations. G2 families were split and each of the two groups exposed to one or the other parasite species. Therefore, we were able to demonstrate that the parasite resistance conferred by the MHC haplotypes did not arise from epigenetic effects as the functional resistance of the haplotypes existed independently of the parasite selecting the G1 fish. An intriguing result of this experiment is the pace at which the resistance alleles increased in frequency. We could show that mortality in G1 did not vary between fish carrying the resistance haplotypes and those lacking it. Thus, the increase in frequency probably arose from more resistant females that produced more clutches. Conversely, females might have also preferred males displaying higher vigour because they possessed those resistance alleles/haplotypes [17] , [27] . Under natural conditions, this adaptive MHC allele frequency shift would lead to reduced prevalence of specific parasites, thus opening the door for other parasites to prevail. Here other MHC alleles would provide resistance and should increase in frequency thereafter. We show that the natural rate of exposure to parasites is sufficient to explain rapid host adaptation (that is, following a single reproductive event), highlighting the evolutionary significance of standing genetic variation. Even though we cannot rule out the possibility that genes in linkage disequilibrium with the detected MHC haplotype were the target of selection, the fact that resistance haplotypes each originated from six different (out of twelve) random wild-caught parents, decreases this likelihood because linkage disequilibrium around these haplotypes should be small. Also, the variation observed at the level of neutral microsatellites suggests that neither demographic changes nor any unobserved type of selection was responsible for the changes in MHC frequencies. Temporal fluctuations of genotypes that are suggestive of Red Queen type dynamics have been demonstrated between invertebrate hosts and their parasites in elegant experimental studies, but the responsible resistance genes were not identified [28] , [29] , [30] , [31] . In our system, however, the resistance genes, that is, MHC class IIβ loci, are known and can be tracked as the genetic target of balancing selection. Hence, our findings have verified an adaptive allele frequency shift, which is indispensable for parasite-mediated selection to directly contribute to the maintenance of MHC polymorphism. Study organism and experimental populations All animal experiments described were approved by the Ministry of Agriculture, Environment and Rural areas in the State of Schleswig-Holstein, Germany. Wild three-spined sticklebacks (parental generation) were collected from a lake (Großer Plöner See, Germany: 54°9′21.16″N, 10°25′50.14″E). To obtain six laboratory-bred families (generation 1, G1), we randomly crossed twelve individuals (parental generation, P). Those G1 fish were split into groups of 20 and raised in the laboratory for 9 months. By randomly assigning 7 males and 7 females per family to each of the 6 experimental ponds, we created 6 populations of equal sex ratio with 84 fish each. The ponds had a capacity of ca. 23 m 3 (3.8×3.8×1.6 m). On one side, the ponds had a shallower part (1 m width×0.5 m depth) to provide male sticklebacks with nesting areas. G1 fish infection Before release into the artificial ponds, the 504 G1 sticklebacks were exposed twice to one of two different parasites. Three laboratory-populations were exposed to the nematode C. lacustris , while the three other populations were exposed to the nematode A. crassus . These two parasites naturally occur in the original host population, and infection success has been shown experimentally to be MHC-dependent [11] . Ripe C. lacustris females were obtained from Eurasian perch ( Perca fluviatilis ) guts whereas A. crassus larvae were isolated from European eel ( Anguilla anguilla ) swim-bladders. Larvae were then counted. Because stickleback infection occurs through trophic transmission, Macrocyclops albidus copepods were bred and infected in the lab. For the first round of fish infection, 6,000 copepods were exposed, in group of 100, to 800 larvae per group that amounts to a total of 48,000 C. lacustris larvae. Identically, we exposed 3,000 copepods to a total of 7,600 A. crassus larvae. The infected copepods were kept during 3 weeks in 1 l tanks to guarantee larvae become infective. This protocol was followed for each copepod infection. To activate the MHC-dependent adaptive immune system of the fish, a second round of infection took place 6 weeks later. We exposed an extra 6,000 copepods to 48,000 C. lacustris larvae and extra 3,000 copepods to A. crassus larvae. Copepod infection was determined by microscopically counting internal nematode larvae. Starved fish were individually exposed to an equal number of infected copepods. Exposure was conducted blind with regard to MHC genotypes of the fish. The fish were then released into the artificial ponds. Egg collection and measurement of parasite resistance During 4 weeks, all egg batches were collected from the ponds and brought to the laboratory. There, a picture of all clutches was taken to estimate the total number of eggs. Every 6 weeks, fish were then counted to measure fish mortality. Twelve weeks after hatching, these G2 clutches were split in groups of twenty fish, reared and exposed to parasites in the same manner as G1 fish. Thirty clutches from G1 were used: half of them originated from the C. lacustris selection treatment while the other half from the A. crassus selection treatment. For each G2 clutch, 15 randomly assigned fish were exposed to C. lacustris , while another 15 were exposed to A. crassus . This resulted in a total of 900 fish to be singly exposed. Again fish were exposed twice to the parasites. For each exposure and parasite, 7,000 lab-bred copepods were isolated and exposed to 57,000 parasite larvae (collected and infected in the same manner as for the G1 generation). For the first exposure, fish received either exactly seven larvae of C. lacustris or exactly nine larvae of A. crassus within the copepods offered. In the second round of infection, the fish were exposed to exactly seven C. lacustris larvae or, owing to a limited availability, randomly from six-to-nine A. crassus larvae in the respective treatment. This exposure resulted in infection levels comparable to that found under natural conditions [17] . In addition, virulence of the parasites could be shown by a negative correlation between parasite load at the end of the experiment and growth during the course of the experiment (for A. crassus , t -value=−3.326, P <0.001; for C. lacustris , t -value=−2.814, P =0.005). Additionally, the fish size at the beginning of the experiment was not correlated with the number of parasites infecting the fish (for A. crassus t -value=1.528, P =0.114; for C. lacustris t -value=−1.622, P =0.106). This suggests that the ones that grew less did so as the result of being infected. DNA extraction and microsatellite typing To record parasite intensity, G1 and G2 fish were dissected following a blindfolded protocol with respect to exposure, that is, fish were checked for both parasites (in the gut and in the swim bladder) 8 weeks after the second exposure. DNA extractions from tail fin tissue were performed using the DNAeasy purification kit (Qiagen) following the manufacturer's protocol. All fish were typed for 18 microsatellites to perform parenthood analysis on the collected clutches [32] . Cloning and MHC typing The 12 wild-caught parental fish were cloned and sequenced for their MHC genotypes. To identify all MHC class IIβ alleles of the exon 2, we cloned and sequenced a fragment spanning from the conserved Exon 1 (GAIIEx1F: 5′-CAG CGT CTC CCT CCT CTT CAT-3′) to the end of Exon 2 (GAIIExon2R_RSCA: 5′-ACT CAC CGG ACT TAG TCA G-3′) of the MHC class IIβ genes, employing cautionary PCR condition,s according to Lenz & Becker [33] . The MHC class IIβ genotypes of the G1 and G2 fish were then determined by reference strand conformation analysis according to Lenz et al . [26] In the population where the parental fish had been caught, certain MHC IIβ sequence variants occur together in haplotype blocks, indicating several gene copies under strong linkage disequilibrium. The number of sequence variants ranges from 1 to 3 among haplotypes either because of a variable number of loci or same alleles on paralogous loci [26] . Furthermore, the stable haplotype organization was confirmed in the present study by the Mendelian segregation of complete haplotypes over two generations. The exon 2 of MHC class IIβ genes was chosen as target gene since it encodes for the peptide-binding groove of the MHC II molecule ( Supplementary Table S1 ). Statistical analyses Statistics were conducted using Primer 6 (ref. 34 ) and the R statistical package [35] . If a selecting parasite increases the frequency of a specific resistance allele, this would be revealed as an increasing proportion of individuals with this allele; therefore, we used proportion as a proxy for frequency. Statistics were conducted in two steps. First, we compared pools of MHC haplotypes between G1 treatments and then between G2 treatments using an ANOSIM on Bray–Curtis similarity matrix with MHC haplotypes as variables. Using a similarity percentage test, we identified haplotypes contributing most to the difference between MHC pools. X 2 tests were used to test for frequency differences of specific haplotype between generations. Our expectations were a haplotype increasing in abundance in a given treatment, for example, C. lacustris , should confer resistance against this parasite [36] . Therefore, we performed a linear mixed effect model with number of parasites (log transformed +1) in G2 fish as dependent variable and G1 treatment, the suspected resistance haplotype (presence versus absence) and zygosity (homozygote versus heterozygote) as fixed effects. Family was a random effect, which accounts for intrinsically linked variation. Tests were conducted on 12 segregating fish families exposed to A. crassus and 13 segregating fish families exposed to C. lacustris . Comparisons were made within fish families so as to evaluate MHC genotype independent from the genomic background. Tests were conducted separately for both G2 treatments ( A. crassus and C. lacustris ). The impact of the suspected resistance haplotypes in G1 were tested similarly with number of parasites (log+1 transformed) as dependent variable and presence of the suspected resistance haplotype and zygosity as predictors. Again, tests were conducted independently for both treatments, the ID of the artificial ponds being used as random factor. How to cite this article: Eizaguirre, C. et al . Rapid and adaptive evolution of MHC genes under parasite selection in experimental vertebrate populations. Nat. Commun. 3:621 doi: 10.1038/ncomms1632 (2012).